Kinetic modelling indicates that fast-translating codons can coordinate cotranslational protein folding by avoiding misfolded intermediates It has been observed for several proteins that slowing down the rate at which individual codons are translated can increase their probability of cotranslational protein folding, while speeding up codon translation can decrease it. Here we investigate whether or not this inverse relationship between translation speed and the cotranslational folding probability is a general phenomenon or if other scenarios are possible. We first derive chemical kinetic equations that relate individual codon translation rates to the probability that a domain will fold, populate an intermediate or misfold, and examine the cotranslational folding scenarios that are possible within these models. We find that speeding up codon translation through misfolding-prone segments can, in some cases, increase the folding probability of a domain immediately before the nascent protein is released from the ribosome and decrease its chances of misfolding. Thus, for some proteins fast-translating codons could be as important as slow-translating codons in coordinating cotranslational protein folding. Cotranslational folding is the process by which a nascent protein domain acquires its folded, tertiary structure during its synthesis by the ribosome [1] . As translation and folding can occur concomitantly, codon translation rates can affect the outcome of the folding process. Indeed, this is exactly what happens in certain cases, as the variability in the rates at which individual amino acids are covalently attached to the C-terminus of the elongating nascent polypeptide chain can strongly influence whether a protein cotranslationally folds and attains its functionality, or misfolds [2] , [3] , [4] , [5] , [6] , [7] . The evidence to date indicates that slowing down translation tends to increase cotranslational folding, and simple arguments suggest that this inverse relationship may be a general phenomenon [8] . Protein folding is a stochastic process, and slower codon translation rates afford a domain extra time to fold during translation. Hence, a common view is that, in the absence of competing processes such as the premature termination of translation [9] , [10] or amino acid misincorporation [11] , slowing translation at specific locations tends to increase the probability of domain-wise cotranslational folding in multidomain proteins, while speeding-up translation tends to decrease it. In this context, a key challenge to understand protein folding in vivo is to develop a framework to model and predict the effects of individual codon translation rates on cotranslational folding, misfolding and intermediate state formation. Such a framework would enable the testing of the range of scenarios that are possible when translation rates are altered, provide an effective tool for analysing in vivo protein-folding experiments, as well as generate a novel systems biology method to predict such behaviour [12] , [13] . It would also have applications in biotechnology by providing a strategy to design mRNA transcripts rationally using synonymous codon mutations that maximize cotranslational folding while simultaneously minimizing misfolding for protein expression protocols [4] , [14] . For all these reasons, a number of studies have examined the role of codon usage across the entire genome of organisms [15] , [16] , [17] . There are several possible approaches to model translation rate effects on cotranslational folding. A particularly straightforward one is to use differential equations in the form of classical chemical kinetic models [18] . Such equations, however, are often difficult to solve analytically for the complex reaction schemes needed to model cotranslational folding. Solving them numerically is possible [19] ; however, with this approach one does not have immediate access to the insights provided by analytical solutions [20] . Alternatively, molecular simulations of the cotranslational folding process can be carried out [21] , [22] . This method is very general; however, one should take into account that even using coarse-grained models it can take many months to simulate the synthesis of a typical protein domain (≈200 residues). An ideal method would, therefore, provide an analytical equation that can predict the probability of cotranslational domain folding ( F ), unfolding ( U ), misfolding ( M ) and intermediate ( I ) state formation ( Fig. 1a,b ) as a function of the rates of translation of individual codons and interconversion between these states and do so without resorting to differential equations. 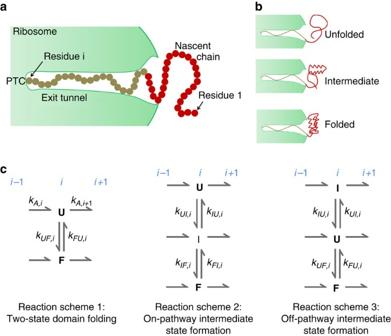Figure 1: Cotranslational folding reaction mechanisms. (a) A schematic cross-section of part of the ribosome exit tunnel through which the nascent chain emerges. PTC, peptidyl transferase centre. A domain (red circles) within the nascent chain has the opportunity to form tertiary structure once it has emerged from the exit tunnel. (b) Three states that a domain may populate during translation are the unfolded, intermediate and folded states. (c) Reaction Scheme 1 corresponds to cotranslational domain folding where no significant population of the intermediate (I) state exists as a result of high folding cooperativity between the folded (F) and unfolded (U) states, whereiis the number of residues in the nascent chain at a given point during its synthesis. Reaction Schemes 2 and 3 correspond, respectively, to situations where a single intermediate state is significantly populated during translation either on or off the pathway to the folded state. Figure 1: Cotranslational folding reaction mechanisms. ( a ) A schematic cross-section of part of the ribosome exit tunnel through which the nascent chain emerges. PTC, peptidyl transferase centre. A domain (red circles) within the nascent chain has the opportunity to form tertiary structure once it has emerged from the exit tunnel. ( b ) Three states that a domain may populate during translation are the unfolded, intermediate and folded states. ( c ) Reaction Scheme 1 corresponds to cotranslational domain folding where no significant population of the intermediate ( I ) state exists as a result of high folding cooperativity between the folded ( F ) and unfolded ( U ) states, where i is the number of residues in the nascent chain at a given point during its synthesis. Reaction Schemes 2 and 3 correspond, respectively, to situations where a single intermediate state is significantly populated during translation either on or off the pathway to the folded state. Full size image Here we use a probabilistic approach to provide such analytical equations [13] , [23] . Within this approach, the probability of taking a particular path through a reaction scheme representing the cotranslational folding of a domain can be exactly computed. In the case of the ribosome, this means that the probability that a nascent protein domain will be in a particular state ( F , U , I or M ) can be calculated as a function of the nascent chain length and the underlying codon translation rates. Using this approach, we examine the process of cotranslational folding and misfolding, and show that fast-translating codons can have an impact on these processes in ways that are unexpected on the basis of current literature. Theoretical methods Our goal is to test whether or not slower translation rates monotonically increase the probability of domain-wise cotranslational folding and examine the relationship between translation speed and intra-domain misfolding. To achieve this goal, we proceed in the following two steps: the first is to derive equations that describe the influence of individual codon translation rates on the cotranslational folding process; the second is to apply to these equations the first derivative test for monotonicity [24] , which tells whether or not slower translation rates monotonically increase the probability of such folding. In this section we address the first step. To formulate equations that can be solved analytically, we make a series of assumptions. First, we assume that the kinetics of the cotranslational folding of a given domain is independent of the folding status of the neighbouring domains [25] . Second, we assume that any domain misfolding or intermediate state formation involves only intra-domain tertiary structure formation. This latter assumption means that the equations resulting from this approach describe only the misfolding of individual domains and cannot be used to describe inter-domain misfolding such as β-strand swapping between two neighbouring domains [26] . Third, we assume that domain folding involves single pathways rather than parallel pathways [27] , [28] . Fourth, we assume that amino-acid addition to the nascent chain is irreversible, as expected under physiological conditions [29] . Fifth, we assume that mistranslation of codons do not occur [11] . Finally, we assume that the elementary reaction steps in the reaction schemes presented below are Markovian [30] , and therefore each state in the reaction schemes is a Markov state. In a previous study we solved a reaction scheme (denoted as RS) representing the cotranslational folding of a domain that can interconvert between only two thermodynamic states, F and U (RS 1 in Fig. 1c ) [13] . Here, we solve reaction schemes that involve an intermediate state that is either on- or off-pathway to the folded state (RS 2 and RS 3 in Fig. 1c ). An off-pathway intermediate is one in which the intermediate cannot directly interconvert with F [31] , while an on-pathway intermediate can do so. In addition, RS 3, in Fig. 1c , can be applied to model intra-domain misfolding by replacing state I with state M . There are up to five unique rates at each nascent chain length in the reaction schemes shown in Fig. 1c . At nascent chain length i , where i is the number of residues comprising the nascent polypeptide chain on an actively translating ribosome, k A, i +1 is the rate at which the i +1 amino acid is covalently attached to the nascent chain; k FU, i and k UF, i are the rates of direct conversion from state F to U and U to F ; k UI, i and k IU, i are the rates of direct conversion from state U to I and state I to U ; and k IF, i and k FI, i are the rates of conversion from state I to F and state F to I . To solve these reaction schemes analytically, we utilize Ninio’s probabilistic approach [23] . Instead of calculating the concentration of a particular species as a function of time, as is traditionally performed in chemical kinetics modelling, in this approach one calculates the probability of taking a particular path along the reaction scheme. With respect to cotranslational folding, we can thus calculate the probability P X ={ F,I,M or U } ,i of a domain being either in state F , I , M or U immediately preceding the addition of the next amino acid to the C-terminus of the nascent chain as a function of the elementary reaction rates ( k A, i , k UF, i , and so on). P X , i is equal to the probability of taking the irreversible path directly connecting states X i and X i +1 , where X corresponds to state F , I , M or U . Thus, this approach yields the probability of being in one of these states as a function of nascent chain length during continuous translation. Within this framework, we have developed a five-step algorithm to determine the equation that relates P X ={ F,I,M or U } ,i to the variety of rates. First, we define the reaction scheme that we wish to solve, as shown in Fig. 1c . Second, we express the probabilities of the various elementary reaction steps in terms of the underlying reaction rates. Third, we use these elementary reaction probabilities to derive the probability of a protein domain taking a particular irreversible path in the reaction when the nascent chain is extended by one residue. Fourth, we determine a compact expression for the recursive relationship between P X , i and P X , i −1 . Finally, we insert the transition probabilities from step three into the recursive relation from step four to yield the analytical solution. To illustrate the use of this algorithm, we derive here an expression for P F, i when a domain can populate an off-pathway intermediate state during biosynthesis ( Fig. 1c , RS 3). To simplify the notation, we denote the elementary reaction probabilities as listed in Fig. 2 , where, for example, a is the probability that, given that a domain is in conformational state I i , it will convert directly to state I i +1 after one step on this reaction scheme. We can write down these elementary reaction probabilities in terms of the underlying reaction rates as shown in Table 1 . This completes Step 2 of our algorithm. 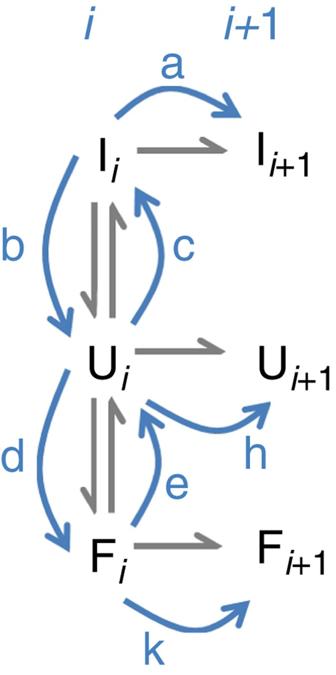Figure 2: Definition of reaction probabilities. The elementary reaction probabilities are indicated by blue arrows and labelleda,b,c,d,e,handkfor the off-pathway intermediate state reaction scheme and can be expressed in terms of the underlying reaction rates (Table 1). Figure 2: Definition of reaction probabilities. The elementary reaction probabilities are indicated by blue arrows and labelled a,b,c,d,e,h and k for the off-pathway intermediate state reaction scheme and can be expressed in terms of the underlying reaction rates ( Table 1 ). Full size image Table 1 Reaction and transition probabilities for the off-pathway reaction scheme. Full size table To determine the transition probabilities (Step 3), we need to calculate the sum of a series representing an infinite random walk at nascent chain length i on this reaction scheme. For example, given that the system starts out in state I i , the probability P ( I i → F i +1 ) that the system will eventually undergo a transition to state F i +1 without first populating states I i +1 or U i +1 , is equal to which corresponds to an infinite series of the form where the binomial term in brackets equals j !/( l ! [ j − l ]!). The sum of the series in Equation 2 is Thus, despite having to account for an infinite random walk through the various thermodynamic states at nascent chain length i , Equation 3 is analytically exact. The transition probabilities for all other possible transitions can be solved in the same manner, and the results of this procedure (see Supplementary Methods ) are listed in Table 1 for RS 3 and Supplementary Tables S1 and S2 for RS 1 and RS 2, respectively. The reaction schemes in Fig. 1c involve a series of irreversible steps, each of which elongates the nascent chain by one residue. As a consequence, the probability of starting out in states F , I or U at nascent chain length i is equal to the probability of being in state F , I or U at length i −1 immediately before the addition of the i th residue to the C-terminus of the nascent chain. Thus, P F, i depends recursively on the events that have taken place at shorter nascent chain lengths [13] . In Step 4 of our approach, we need to solve a compact form of this recursive relation for P F, i . To obtain this solution, we first note that We emphasize again that at nascent chain length i the initial probabilities of being in state F , I or U are equal to P F, i −1 , P I, i −1 and P U, i −1 , respectively, and these terms are therefore constants in Equation 4. This equation enables us to calculate the contributions of these initial probabilities to the final probability P F, i of being in state F immediately before adding the i +1 residue. A compact form of the recursive relation, from i =1 residues up to N residues, can be obtained by writing down Equation 4 for the specific cases of i =1, 2 and 3, noting that the initial conditions for the ribosome nascent chain complex are P F,0 =0, P I,0 =0 and P U,0 =1 (that is, the initial probability of the domain being unfolded equals unity when the nascent chain is one residue in length), and searching for a pattern. The pattern that emerges from this procedure can be written as A detailed derivation of Equation 5 is provided in the Supplementary Methods . Equation 5 expresses the influence of the transition probabilities, starting from the incorporation of the first amino acid into the P-site of the ribosome, on the probability of the domain being folded at nascent chain length i immediately before addition of the i +1 residue. We note that Equations 4 and 5 can also potentially be derived using dynamic programming methods [32] . Inserting the elementary reaction probabilities ( Table 1 ) into Equation 5, which is Step 5 in our algorithm, yields the analytic solution of P F, i in terms of the elementary reaction rates k A, i , k UF, i , k UI, i , k UI, i and k IU, i For the sake of compactness, we have inserted the variable D j into Equation 6 where D j =[ k A, j +1 + k IU, j ][ k A, j +1 + k FU, j + k UF, j ]+ k UI, j [ k A, j +1 + k FU, j ]. This algorithm can be applied to solve for P U, i , and to the other reaction schemes shown in Fig. 1c in order to obtain their analytical solutions. The effect of translation rates on folding The use of the theoretical approach that we have presented above enables us to obtain the probabilities of a domain being in states F, I, M or U during continuous translation as a function of the nascent chain length and the elementary reaction rates ( Table 2 ). RS 1, which was solved previously [13] , models one of the simplest possible types of cotranslational behaviour, in which a domain can reversibly fold and unfold in an apparent two-state manner. RS 2 and RS 3 are more general, as they account, respectively, for the situation where on- and off-pathway intermediate states are formed during translation. Thus, these analytical solutions are able to model codon translation rate effects on important types of cotranslational protein behaviour involving single pathway domain folding. Table 2 Folding-state probabilites during nascent chain extension. Full size table Fast translation can increase folding of two-state domains The analytical solutions in Tables 1 and 2 allow us to determine the scenarios that are possible when codon translation rates are altered, and thereby to test theoretically if in general, slower translation rates increase monotonically the probability of cotranslational folding. Of particular interest is whether or not there are any unconventional situations in which the probability of cotranslational folding can be decreased by slowing down codon translation rates, and increased when the speed of translation is increased. We first consider domains that can be modelled as folding in a two-state manner ( Fig. 1c , RS 1), and ask how decreasing k A, i +1 (that is, slowing down translation) changes the cotranslational folding probability immediately before the nascent chain is released from the ribosome: does it increase P F, i , decrease P F, i or exhibit more complex behaviour depending on the other rates? The equation in Table 2 allows us to determine mathematically which of these scenarios occurs by applying the first derivative test for monotonicity [24] . That is, if we were to take the derivative of the P F, i equation for RS 1 in Table 2 with respect to k A, i +1 , holding the other rates constant, and find that the derivative is less than or equal to zero for all possible values of k A, i +1 , k UF, i and k FU, i , then slowing down the translation rate of a codon (or group of codons) will always cause P F, i to increase or remain equal to its value before the decrease in the codon translation rate; in this case, P F, i is monotonically decreasing. By contrast, if this derivative is greater than, or equal to, zero for all possible values of k A, i +1 , k UF, i and k FU, i then P F, i is monotonically increasing with the translation rate; that is, slower translating codons will always decrease the cotranslational folding probability or at least keep it constant. Alternatively, if the derivative is positive for some values of the rates and negative for others then P F, i is non-monotonic with respect to k A, i +1 . In this case, decreasing the translation rate of a given codon may either increase or decrease the probability of cotranslational domain folding depending on the behaviour of k UF, i and k FU, i as a function of nascent chain length; a result that would be contrary to the conventional view that this derivative should always be negative. In addition to being able to apply this monotonicity test to the equations in Table 2 , we can also apply this test to Equation 4 without any loss of generality. The advantage of using Equation 4, which is applicable at all nascent chain lengths, is that the relationship of P F, i to the transition probabilities is notationally much simpler. Therefore, we have applied the first derivative test to this equation and, since we are considering a domain that cannot populate an intermediate state P I, i −1 =0 at all nascent chain lengths and Equation 4 reduces to Inserting the transition probabilities for RS 1 ( Supplementary Table S1 ) into Equation 4 we have where P F, i −1 and P U, i −1 are constants, as noted in the Theoretical Methods section. Therefore, the partial derivative of Equation 8 with respect to k A, i +1 is The range of possible values of k A, i +1 , k UF, i and k FU, i are in the interval [0,∞]. The denominator in Equation 9 is therefore always positive, while the numerator can be either positive or negative. Thus, for two-state domain folding P F, i is non-monotonic as a function of the codon translation rates. We can gain insight into the situations where P F, i increases or decreases with changes in translation rate by noting that the constant P F, i −1 can be expressed in terms of the equilibrium folding probability , at nascent chain length i , as P F, i −1 = c i , where c i is a constant of proportionality. can in principle be measured on a ribosome that has been arrested indefinitely at nascent chain length i [33] , [34] . The proportionality constant c i is <1 when P F, i −1 < , and c i >1 when P F, i −1 > . is a function of the elementary reaction rates and is equal to = k UF, i /[ k UF, i + k FU, i ]; therefore, P F, i −1 = c i k UF, i /[ k UF, i + k FU, i ]. Inserting the latter equation into Equation 9 we have With the derivative expressed in these terms it is easier to interpret its physical meaning. When P F, i −1 < the derivative is negative, and when P F, i −1 > the derivative is positive. Therefore, at nascent chain length i , if the initial domain-folding probability (immediately after adding the i th residue to the nascent chain) is less than its equilibrium value at length i , then c i <1 and decreasing the translation rate of codon i +1 will monotonically increase the probability of cotranslational domain folding. Equivalently, increasing k A, i +1 will monotonically decrease P F, i . If, however, the initial domain-folding probability is greater than its equilibrium value then decreasing the translation rate of codon i will monotonically decrease the probability of cotranslational domain folding. The equilibrium probability , which influences the sign of ∂ P F, i /∂ k A, i +1 through Equation 10, is a function of the free energy of domain stability, Δ G FU,i , of F relative to U as expressed by the equation . Therefore, a pertinent question is to ask what trends in Δ G FU ,i with nascent chain length can cause c i to be greater than or less than 1, and consequently the derivative in Equation 10 to be either positive or negative. We find that if Δ G FU ,i is a monotonically decreasing function of nascent chain length i (illustrated in Fig. 3a,b , top panel)—that is, if the folded domain becomes progressively more stable—then the derivative is negative and slowing down translation can increase the cotranslational folding probability before the nascent chain is released from the ribosome ( Fig. 3c ), while speeding up translation can decrease this final folding probability. This result is consistent with the conventional view that slowing down translation should promote cotranslational folding. Another scenario, however, also exists according to these equations; if the domain stability changes non-monotonically with nascent chain length ( Fig. 3a,b , bottom panel), being stable at some lengths but unstable at others, then c i can be positive at some nascent chain lengths. This means that speeding-up translation can monotonically increase the probability that a two-state domain will cotranslationally fold and slow-translating codons can decrease folding. In this case, we find that speeding up translation through destabilizing regions maximizes cotranslational folding ( Fig. 3d ). These examples illustrate a mechanistic way in which fast-translating codons can enhance the cotranslational folding of domains that fold in a two-state manner, a result that is unexpected based on the current literature. 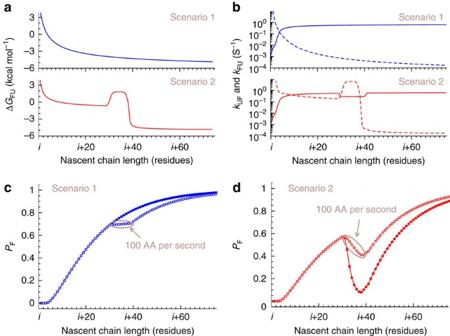Figure 3: The effect of fast-translating codons on two-state folding. Scenarios 1 and 2 are two different types of behaviour exhibited by Reaction Scheme 1. (a) Equilibrium stability of folded and unfolded states as a function of nascent chain length illustrated using hypothetical data. In Scenario 1, the folded-state stability monotonically changes with nascent chain length, and in Scenario 2 a non-monotonic change occurs. (b) Folding and unfolding rates as a function of nascent chain lengths for Scenarios 1 and 2 that give rise to the stability curves ina. The folding rate,kUF, and unfolding rate,kFU, are shown, respectively, as solid and dashed lines. (c) Predicted cotranslational domain-folding probability as a function of nascent chain length for Scenario 1, using the rates frombas arguments in the equation for RS 1 inTable 2. In one example, the ribosome translates each codon with a rate of 10 AA per second (solid blue squares); in the other example, translation of codonsi+31 throughi+39 is increased up to a hypothetical 100 AA per second (open blue circles), while the codons outside this region translate at 10 AA per second.dreflectsc, except using Scenario 2. Note that when the fast-translating codons are inserted into the mRNA, the final folding probability at nascent chain lengthi+75 residues is decreased slightly in Scenario 1 (c) and increased in Scenario 2 (d). Figure 3: The effect of fast-translating codons on two-state folding. Scenarios 1 and 2 are two different types of behaviour exhibited by Reaction Scheme 1. ( a ) Equilibrium stability of folded and unfolded states as a function of nascent chain length illustrated using hypothetical data. In Scenario 1, the folded-state stability monotonically changes with nascent chain length, and in Scenario 2 a non-monotonic change occurs. ( b ) Folding and unfolding rates as a function of nascent chain lengths for Scenarios 1 and 2 that give rise to the stability curves in a . The folding rate, k UF , and unfolding rate, k FU , are shown, respectively, as solid and dashed lines. ( c ) Predicted cotranslational domain-folding probability as a function of nascent chain length for Scenario 1, using the rates from b as arguments in the equation for RS 1 in Table 2 . In one example, the ribosome translates each codon with a rate of 10 AA per second (solid blue squares); in the other example, translation of codons i +31 through i +39 is increased up to a hypothetical 100 AA per second (open blue circles), while the codons outside this region translate at 10 AA per second. d reflects c , except using Scenario 2. Note that when the fast-translating codons are inserted into the mRNA, the final folding probability at nascent chain length i +75 residues is decreased slightly in Scenario 1 ( c ) and increased in Scenario 2 ( d ). Full size image Fast translation can minimize the misfolded population While small proteins that fold in an apparent two-state manner have been the focus of many in vitro protein-folding studies [35] , the majority of naturally occurring proteins, by virtue of their larger size, are likely to fold through a series of intermediates [36] , [37] , [38] , populating stable on- or off-pathway intermediates besides the folded and unfolded states. An important question then concerns how altering codon translation rates affects these proteins. To answer this question we again apply the first derivative test. In this case, however, we use the transition probabilities listed in Table 1 and insert them into Equation 4. For the situation in which an off-pathway intermediate state can form ( Fig. 1c , RS 3), the first derivative of P F, i with respect to k A, i +1 is proportional to For the sake of clarity in Equation 11 we have presented only the factors that determine the derivative in terms of k A, i +1 ; we provide the exact expression in Supplementary Eq. S22 . As all the elementary rates must be in the interval [0,∞] the first term in Equation 11 is always positive, the second term always negative and the third term is either positive or negative depending on the rates other than k A, i +1 . Therefore, these terms make opposing contributions to the sign of the derivative. Adding these terms together means that ∂ P F, i /∂ k A, i +1 can be either negative or positive depending on the values of the various rates, and P F, i is therefore a non-monotonic function of k A, i +1 . Thus, for cotranslational folding domains that can populate an off-pathway intermediate state, or an intra-domain-misfolded state, faster-translating codons can in some cases increase the cotranslational domain-folding probability immediately before release of the nascent protein from the ribosome and decrease it in others. To illustrate this point, consider the hypothetical example of a multidomain protein containing a large domain of predominantly α-helical structure, which during synthesis can populate an off-pathway intermediate (or misfolded) state involving the formation of non-native tertiary structure localized in the region of the domain that is closest to the N-terminus of the nascent chain ( Fig. 4 ). If synthesis is very slow, then the first part of this domain will emerge from the ribosome exit tunnel before the second half and will therefore have a significant amount of time to assemble into this non-native structure. When the second part of the domain finally emerges from the exit tunnel it will not be able to assemble into the fully folded domain structure until the non-natively structured intermediate first unfolds. In this example, slowing down translation can decrease the probability of cotranslational folding. If the domain were to be synthesized rapidly then a smaller population of the off-pathway intermediate would be present once the complete sequence of the domain had emerged from the exit tunnel; therefore, the domain could fold more rapidly into its native structure because it would not need to wait for the unfolding of the intermediate. 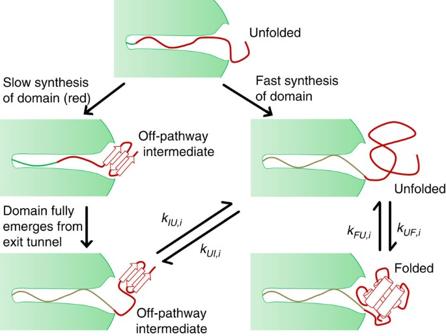Figure 4: Fast-translating codons increasing cotranslational folding. For such a domain (shown in red), slow-translation rates (left hand side) can allow for the accumulation of the off-pathway intermediate before the full-length segment comprising the domain has emerged from the exit tunnel. This effect can delay cotranslational folding because the intermediate must unfold in order for the domain to reach its folded state. In contrast, fast synthesis of the domain (right hand side) can minimize the population of the off-pathway intermediate and allow the domain to partition quickly into the folded state. Figure 4: Fast-translating codons increasing cotranslational folding. For such a domain (shown in red), slow-translation rates (left hand side) can allow for the accumulation of the off-pathway intermediate before the full-length segment comprising the domain has emerged from the exit tunnel. This effect can delay cotranslational folding because the intermediate must unfold in order for the domain to reach its folded state. In contrast, fast synthesis of the domain (right hand side) can minimize the population of the off-pathway intermediate and allow the domain to partition quickly into the folded state. Full size image Numbers are put to this scenario in Fig. 5 where hypothetical data are utilized that represent realistic values of typical folding and unfolding rates [12] , [39] . The results in Fig. 5 indicate that when any off-pathway intermediate, regardless of its structural details, becomes thermodynamically stable at nascent chain lengths shorter than that at which the full domain becomes stable (Scenario 4 in Fig. 5a,b ), then speeding up translation can increase the final cotranslational folding probability ( Fig. 5c ). Conversely, if the intermediate was only to form in the second part of the domain, closer to the C-terminus (Scenario 3 in Fig. 5a,b ), then slowing down translation can monotonically increase the final cotranslational folding probability ( Fig. 5d ). 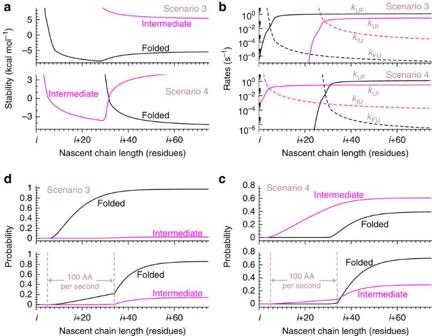Figure 5: Effect of fast-translating codons on an off-pathway intermediate. Scenarios 3 and 4 are two different types of behaviour exhibited by Reaction Scheme 3. (a) Equilibrium stability of the folded and intermediate states of a protein domain as a function of nascent chain length. Two scenarios are possible on an arrested ribosome: in Scenario 3, the folded state of the domain becomes thermodynamically stable at shorter lengths than the intermediate, and in Scenario 4 the opposite situation occurs. (b) Rates of interconversion between states F, I and U as a function of nascent chain lengths for Scenarios 3 and 4 that give rise to the stability curves ina. (c) Probability of populating F or I as a function of nascent chain lengths for Scenario 4. In the top panel, all codons are translated at the same rate of 10 AA per second; in the bottom panel, the translation of codonsi+5 throughi+35 are increased in rate up to a hypothetical 100 AA per second. (d) reflects (c), except using Scenario 3. In contrast to Scenario 3, Scenario 4 shows that speeding up translation can increase the final cotranslational folding probability (bottom versus top panel of (c)). Figure 5: Effect of fast-translating codons on an off-pathway intermediate. Scenarios 3 and 4 are two different types of behaviour exhibited by Reaction Scheme 3. ( a ) Equilibrium stability of the folded and intermediate states of a protein domain as a function of nascent chain length. Two scenarios are possible on an arrested ribosome: in Scenario 3, the folded state of the domain becomes thermodynamically stable at shorter lengths than the intermediate, and in Scenario 4 the opposite situation occurs. ( b ) Rates of interconversion between states F, I and U as a function of nascent chain lengths for Scenarios 3 and 4 that give rise to the stability curves in a . ( c ) Probability of populating F or I as a function of nascent chain lengths for Scenario 4. In the top panel, all codons are translated at the same rate of 10 AA per second; in the bottom panel, the translation of codons i +5 through i +35 are increased in rate up to a hypothetical 100 AA per second. ( d ) reflects ( c ), except using Scenario 3. In contrast to Scenario 3, Scenario 4 shows that speeding up translation can increase the final cotranslational folding probability (bottom versus top panel of ( c )). Full size image The intra-domain misfolding of a protein can also be modelled using the off-pathway reaction scheme in RS 3 in Fig. 1c , where I is replaced by state M . Therefore, the conclusions drawn above also apply to intra-domain misfolding. Understanding the process by which proteins fold during their biosynthesis is one of the most fundamental problems in molecular biology, as it is crucial to enable their biological function [3] , [40] , and its failure can result in their misfolding [40] , [41] , [42] , malfunction [7] and aggregation [3] , [4] , [43] , events that are associated with a wide range of severe health conditions including neurodegenerative disease [44] . A key challenge in this context is to interpret and predict the influence of individual codon translation rates on cotranslational protein folding and misfolding. The benefits of responding to this challenge are manifold: it would provide models with which to interpret high-resolution experiments [33] , [34] ; it would allow the results obtained from studies of nascent chains attached to ribosomes arrested in the process of protein synthesis to be utilized to predict nascent protein behaviour during continuous translation [13] ; it would offer insights into codon usage bias across the transcriptomes of different organisms [45] ; and it would provide a better understanding of the variety of folding and misfolding events that are possible during continuous translation [1] . In the present study, we have derived two equations ( Table 2 ) that describe the influence of individual codon translation rates on cotranslational folding involving pathways in which on- and off-pathway intermediates can form. These equations, which depend on the underlying codon translation rates, provide a framework to integrate data from measurements performed on arrested RNCs, where k A, i +1 =0, and make predictions that are testable by a range of experimental techniques including NMR [33] and single molecule [34] methods. Recently, for example, T4–lysozyme was identified as folding on the ribosome with an on-pathway intermediate, and the rates k UI, i , k IU, i and k IF, i were measured at two different nascent chain lengths [34] . If measurements of these rates at more nascent chain lengths were carried out, they could be used as arguments in the on-pathway reaction scheme equation in Table 2 to predict how the populations F , I and U are influenced by individual codon translation rates. These equations provide a means of testing the general idea that slowing translation will monotonically increase the probability that a domain will fold cotranslationally, and conversely that speeding up translation will decrease this probability [2] , [3] , [4] , [5] , [6] . In this work, we have tested this idea by analysing the dynamic behaviour of these cotranslational folding models, and indeed we have found that there are situations in which other scenarios are possible. These are situations in which slowing down translation can actually decrease the final cotranslational folding probability of a domain immediately before the nascent chain is released from the ribosome. Stated in a different but equivalent form, there are situations in which speeding up the rate at which segments of a protein are synthesized will increase the final probability of cotranslational folding and decrease the probability of intra-domain misfolding. For a domain that folds in a two-state manner, this situation can arise when its stability in the folded state exhibits non-monotonic changes with nascent chain length. For example, in Fig. 3a (Scenario 2) the folded state of a ribosome-bound domain becomes progressively more thermodynamically stable as the nascent chain elongates. Between nascent chain lengths i +30 and i +38, however, it becomes less stable, and beyond these lengths the folded state again becomes more stable. We have demonstrated, using the rates shown in Fig. 3b and equation RS 1 in Table 2 , that speeding up translation along this destabilizing stretch of nascent chain increases the final folding probability ( Fig. 3d ), and that slowing translation decreases this probability. In contrast to this result, in Scenario 1 shown in Fig. 3 , where the folded state becomes progressively more stable with nascent chain length, we have found that slowing translation monotonically increases the final cotranslational folding probability ( Fig. 3c ). Thus, even for domains exhibiting the simplest possible folding behaviour on the ribosome, slow-translating codons can in certain circumstances affect cotranslational behaviour in different ways depending on the context. We note in addition the interesting result that molecular chaperones, such as trigger factor [46] , can serve as a cause of non-monotonic changes in domain stability [47] because of their binding to the unfolded ensemble [46] . A similar result was found for domains that can populate an off-pathway intermediate or an intra-domain-misfolded state during cotranslational folding. In this case, however, this behaviour is not caused by non-monotonic changes in stability, but rather it is the balance between the nascent chain length at which the intermediate becomes thermodynamically stable relative to that when the folded domain becomes stable. In cases where the folded domain becomes more stable at shorter nascent chain lengths than the intermediate, slowing translation can monotonically increase the final probability of folding (Scenario 3 in Fig. 5 ). When, however, the intermediate becomes stable before the complete domain has emerged from the exit tunnel, slowing translation can decrease the final probability of folding (Scenario 4 in Fig. 5 ) and fast codons can increase it. These results therefore indicate that there is much greater complexity in the possible effects of codon translation rates on folding than one might have expected. For example, replacement of rare codons with common codons, which are presumed to be translated more quickly, has been found to decrease the cotranslational folding of a number of proteins [2] , [6] , [40] , and an in vivo assay examining heterologous protein expression found that four different proteins exhibited increased cotranslational folding when translation rates were globally decreased using a streptomycin-sensitive Escherichia coli strain [3] . The predictions made in the present study indicate that exceptions can exist, and we hope these results will motivate experimental investigations to search for nascent proteins that exhibit increased cotranslational folding upon an increase in individual codon translation rates. We anticipate that protein molecules that may exhibit such behaviour are more likely to be multidomain proteins containing at least one domain that is known to populate an off-pathway intermediate state in vitro involving the N-terminal portion of the protein. The cotranslational folding scenarios and conclusions presented here are robust as they are based on the derivatives of the mathematical models given in Table 2 with respect to codon translation rates, rather than specific values for these rates. Derivatives of these models characterize the dynamic scenarios that are possible when arbitrary changes are made to the codon translation rates. Furthermore, as we have described, the simplest mechanisms of cotranslational folding (that is, two-state and three-state mechanisms) exhibit the scenario that fast-translating codons can be beneficial to folding; it therefore seems likely that cotranslational mechanisms of even greater complexity will also exhibit such behaviour. It has been proposed previously that fast-translating codons can help to avoid protein misfolding [11] , although through a fundamentally different mechanism than the one we have identified. The mistranslation-induced protein-misfolding hypothesis posits that fast-translating codons (that is, optimal codons) minimize misfolding by avoiding mistranslation, and therefore evolution has selected for optimal codons in highly expressed proteins to avoid the cellular burden of dealing with a large number of proteins driven to misfold because of mutations in their primary structure [48] , [49] . Our results suggest that even in the absence of mistranslation, fast-translating codons can still have a biologically important and advantageous role to play by minimizing the chances that a protein will misfold. Teasing out the relative contribution of each of these mechanisms to mRNA sequence evolution will help us understand better the forces shaping the cotranslational folding landscape of the proteomes of different organisms. Our results have implications for the evolution of mRNA sequences and of biases in the codon usage in the transcriptomes of different organisms [50] . Early studies examining synonymous codon usage in mRNA sequences and their correlations with a small number of domain structures found some evidence that rare codons are more frequently used at or near domain boundaries [14] , [51] , [52] , suggesting that these codons are likely to be translated more slowly to provide a domain with more time to fold into its correct structure, thus avoiding misfolded states [1] . A more extensive analysis across a large number of transcriptomes and proteomes found, however, no evidence for such a correlation [45] . Our results suggest that this absence of a proteome-wide correlation between domain boundaries and slow codons could arise when both fast- and slow-translating codons, used in different contexts, increase the overall folding probability of domains ( Fig. 6 ). Domains whose stability in the folded state progressively becomes greater with nascent chain length may benefit from having mRNAs that contain slow-translating codons near their domain boundaries, while domains that exhibit non-monotonic changes in stability or populate off-pathway intermediates may benefit from stretches of fast-translating codons. If such behaviour is evenly distributed across the transcriptome, then the correlation between codon usage and domain boundaries would cancel out upon averaging over the entire proteome. 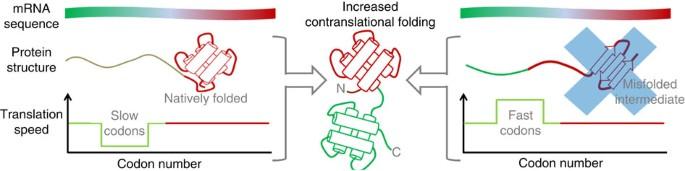Figure 6: Fast- and slow-translating codons can increase cotranslational folding. If a domain folds without populating intermediates at significant levels then a stretch of slow-translating codons near the domain boundary can increase folding (left hand side). If a segment of a domain can populate an off-pathway intermediate then by rapidly translating that segment can increase the probability of cotranslational folding (right hand side) by helping avoid the misfolded intermediate (blue X). Figure 6: Fast- and slow-translating codons can increase cotranslational folding. If a domain folds without populating intermediates at significant levels then a stretch of slow-translating codons near the domain boundary can increase folding (left hand side). If a segment of a domain can populate an off-pathway intermediate then by rapidly translating that segment can increase the probability of cotranslational folding (right hand side) by helping avoid the misfolded intermediate (blue X). Full size image A prediction based on our results is that fast-translating codons may be more frequently found in misfolding-prone domains than those domains that fold cooperatively, that is, without significantly populated intermediates. We note, however, that proteins that can misfold during translation in their native environment have not yet been experimentally identified; therefore, we do not at present have an accurate data set to test this hypothesis. We therefore created a surrogate data set by looking for enrichment of fast codons in large domains (>200 residues in size), which we assumed were likely to misfold relative to small domains (<90 residues), which we assumed would not misfold. Using three different metrics to define fast codons (codon abundance, the Codon Information Index [53] and Barral’s Method [4] ), we found no statistically significant difference between these two groups in E. coli (data not shown). However, just as the lack of a proteome-wide enrichment of slow codons at domain boundaries [45] does not mean that slow codons do not have a significant impact [5] , it is also possible that fast-translating codons can increase folding for some proteins despite a lack of enrichment when averaged across many proteins. It is more likely, however, that the data set we have used is simply insufficient to test our hypothesis. In the future, as cotranslationally misfolded proteins are identified experimentally, it will be important to revisit this analysis. Circumstantial experimental evidence that both fast- and slow-translating codons could potentially be utilized to increase the probability of cotranslational folding comes from bioinformatic studies at the protein secondary-structure level, rather than the domain level, and also from the field of biotechnology. Two bioinformatic studies recently explored that correlation between codon usage with protein structure using different metrics to define codon optimality. In the first study, it was found that protein structure-containing coils are translated more quickly than α -helical or β -strand structures [45] . In the other study, it was found that both optimal and non-optimal codons are enriched in α -helical and β -strand structures [16] . These results are consistent with the notion that both fast- and slow-translating codons play a role in coordinating cotranslational folding; however, they do not rule out alternative hypotheses of their functional consequences. Advances in biotechnology are shedding light on the importance of fast-translating codons in the coordination of cotranslational folding. In heterologous protein expression, a gene from an organism (the genetic source) is inserted into an organism of a different species (the host) for the purpose of expressing the protein encoded by the gene. Owing to the degeneracy of the genetic code (61 codons encoding for the 20 naturally occurring amino acids), there is an astronomically large number of possible mRNA sequences that encode for the same protein sequence. Therefore, an important challenge in heterologous protein expression is designing an mRNA sequence using fast- or slow-translating synonymous codons that maximizes the yield of soluble folded protein product. The Codon Optimization (CO) method designs such an mRNA sequence by utilizing the host’s most frequently used synonymous codons at each codon position along the designed mRNA sequence. The Codon Harmonization (CH) method, on the other hand, designs an mRNA sequence to reproduce in the host organism the original codon usage pattern found in the genetic source [54] . In the case of the protein firefly luciferase, expressed in E. coli , the CO- and CH-designed mRNA sequences yield similar average translation rates, as reported in Spencer et al . [4] The CH-designed mRNA sequence, however, produces a larger variation in the translation speed, with more fast- and slow-translating segments contained in its open reading frame. This greater variation in translation speed apparently results in the larger fraction of folded luciferase when compared with the situation with the CO-designed sequence [4] . This finding is consistent with the results presented in this work as it suggests that it is possible that the larger number of fast-translating codons in the CH-designed mRNA sequence contributes to the observed increase in the fraction of folded luciferase. The cotranslational folding scenarios that we have analysed in this study involve single pathways ( Fig. 1c ), yet parallel pathways have been observed in vitro [27] , [28] and are expected to occur for many proteins based on statistical mechanical models [55] and molecular dynamics simulations of protein folding [56] . An important extension of the present study will be to derive a general formalism to solve analytically for arbitrarily complex cotranslational folding reaction schemes in which multiple intermediate states can be populated, and those states can all interconvert directly with one another. Such a formalism would allow parallel cotranslational folding, inter-domain interactions and inter-domain misfolding pathways to be modelled explicitly for both cytosolic and membrane proteins. Analytical solutions to reaction schemes have heavily influenced the way in which in vitro protein-folding experiments are analysed [57] and how protein folding is understood at the molecular level [58] , [59] . Such approaches have also been successful in modelling the competition between protein misfolding and aggregation [20] , [60] . The approach presented here represents an extension of such reaction schemes to reflect the multiplicity of folding and misfolding processes occurring within a cell. With the recent application of highly accurate spatial- and time-resolved experiments of cotranslational folding [34] , [61] we believe that the quantitative models that we have presented here will offer novel opportunities for interpreting, understanding and predicting the earliest events in in vivo protein folding. How to cite this article: O’Brien, E. P. et al . Kinetic modelling indicates that fast-translating codons can coordinate cotranslational protein folding by avoiding misfolded intermediates. Nat. Commun. 5:2988 doi: 10.1038/ncomms3988 (2014).